ArabidopsisAZI1 family proteins mediate signal mobilization for systemic defence priming Priming is a major mechanism behind the immunological ‘memory’ observed during two key plant systemic defences: systemic acquired resistance (SAR) and induced systemic resistance (ISR). Lipid-derived azelaic acid (AZA) is a mobile priming signal. Here, we show that the lipid transfer protein (LTP)-like AZI1 and its closest paralog EARLI1 are necessary for SAR, ISR and the systemic movement and uptake of AZA in Arabidopsis . Imaging and fractionation studies indicate that AZI1 and EARLI1 localize to expected places for lipid exchange/movement to occur. These are the ER/plasmodesmata, chloroplast outer envelopes and membrane contact sites between them. Furthermore, these LTP-like proteins form complexes and act at the site of SAR establishment. The plastid targeting of AZI1 and AZI1 paralogs occurs through a mechanism that may enable/facilitate their roles in signal mobilization. Plants recognize pathogens via perception of conserved molecular patterns from microbes (MAMPs; microbe-associated molecular patterns), such as flg22 peptides from bacteria flagellum, or effectors that microbes use to suppress plant defences [1] . After recognition, local and systemic immunity are established [2] . Plants induced for systemic immunity show broad spectrum and long-lasting resistance to new infections [3] . Systemic resistance involves an energy-saving ‘primed state’, such that secondary infections of distal leaves induces a faster and/or stronger defence than occurs in naive plants [4] . Different types of systemic defence programs are established depending on the inducing microbe, as well as the plant tissue where local immunity is triggered [5] . When a pathogen or MAMP is recognized in leaves, plants induce systemic acquired resistance (SAR) or MAMP-triggered SAR (mSAR) [6] , [7] . However, if a first exposure occurs in the roots, usually with a beneficial microbe, plants trigger induced systemic resistance (ISR). Although SAR and ISR result in a similar level of pathogen resistance, few common components are known to be shared [5] , [8] . Only a handful of factors specifically affect SAR without affecting local disease resistance [9] , [10] , [11] , [12] , [13] . These SAR-specific components are candidates for generating/mobilizing and/or being receptors for mobile signals. On the other hand, many natural priming signals have been proposed, including azelaic acid (AZA) and its precursor/derivatives, methyl salicylate, jasmonic acid, dehydroabietinal, pipecolic acid and a glycerol-3-phosphate-dependent metabolite [10] , [12] , [14] , [15] , [16] , [17] , [18] , [19] . The existence of more than one signal capable of establishing a primed state suggests that plants may use a consortium of molecules to reach a certain ‘priming threshold’. Responses to specific signals can depend on plant growth/infection conditions, which highlights the plasticity of plant responses [10] , [14] , [16] , [20] , [21] , [22] . A key unexplored aspect of systemic resistance/priming establishment is the process by which the signal(s) are mobilized from the site of cellular synthesis to the vascular stream, where they are moved and finally taken up by the distal cells. Plants can move small proteins and metabolites to systemic tissues mainly using the phloem [23] . Because uploading to the phloem can be apoplastic and/or symplastic, signals must reach the endoplasmic reticulum (ER)–plasmodesmata and/or the apoplast. Soluble signals can move freely once they reach the cytoplasm, but hydrophobic signals require a specific transport mechanism. In the case of SAR-inducing petiole exudates, the main biologically active fraction is apolar [19] . Thus, movement of SAR signals must involve deployment of transport machineries. Intracellular transport of lipidic molecules could use vesicular or non-vesicular transport through transporter/chaperone proteins as well as by direct membrane–membrane contact (membrane contact sites; MCSs) [24] , [25] . In plants, MCSs occur between the chloroplast, ER and plasma membrane (PM) [26] , [27] . Lipid transfer proteins (LTPs) are key components in MCS formation, where lipid exchange occurs [27] , [28] , [29] . Two of the few known SAR-specific components are azelaic acid induced 1 (AZI1) and defective in induced resistance 1 (DIR1) [10] , [11] . Both proteins have eight cysteine motifs (8CM) commonly associated with LTPs and have one or more paralogs. AZI1 and DIR1 belong to different families: the hybrid proline-rich proteins (HyPRPs) and the non-specific LTPs [30] , respectively. Mutants of AZI1 and DIR1 not only lack SAR, but are also either locally ( dir1 ) or systemically ( azi1 ) non-responsive to the AZA mobile priming signal, a lipidic 9 carbon dicarboxylic acid [10] generated from plastid galactolipid oxidation during infection [22] , [31] . Full dehydroabietinal responsiveness also requires DIR1 and AZI1 and is enhanced in the presence of AZA [17] . DIR1 and AZI1 were proposed to form part of a functional unit [12] , [32] and can form complexes that localize to the ER and plasmodesmata [32] . This work reveals novel localization to plastids, strong membrane association properties and previously undescribed signalling functions for AZI1 and its close paralog early Arabidopsis aluminium induced 1 (EARLI1), which are needed for moving AZA/AZA derivative(s) and establishing SAR, mSAR and ISR. In addition, we give the first evidence for a specific function of the proline-rich region (PRR) of AZI1 and related proteins as a component of a plastid-targeting signal that is likely a general property of many HyPRPs in the plant kingdom. A pool of AZI1 localizes to chloroplast outer envelopes To gain insight into how AZI1 and DIR1 might differ in their contribution to SAR and AZA-induced priming, we studied the locations in Nicotiana benthamiana of dexamethasone (Dex)-inducible green fluorescent protein (GFP) fusion proteins within cells. The control, soluble GFP, was distributed uniformly in the cytosol and nucleus ( Supplementary Fig. 1a ). GFP patterns of AZI1:GFP and DIR1:GFP were consistent with plasmodesmata (punctate structures at cell peripheries maintained after plasmolysis), PM and ER network ( Fig. 1a , Supplementary Fig. 1b ), in agreement with Yu et al . [32] . AZI1:GFP was also visible in ER transcytoplasmic strands and ring patterns similar to outer envelope membrane (OEM) proteins that tightly surrounded chloroplasts [33] and in stromule-like projections ( Fig. 1a,b ). This chloroplastic pattern was also observed when AZI1:GFP levels were lower (driven by constitutive 35S promoter; Supplementary Fig. 1c ). AZI1:GFP co-localized with the OEM marker OEP7:RFP (red fluorescent protein) around chloroplasts and partially with BiP:RFP, an ER marker, in contact sites between ER and chloroplast/stromules ( Fig. 1c ). In contrast, DIR1:GFP co-localized only with BiP:RFP and was not found around chloroplasts ( Fig. 1d ). 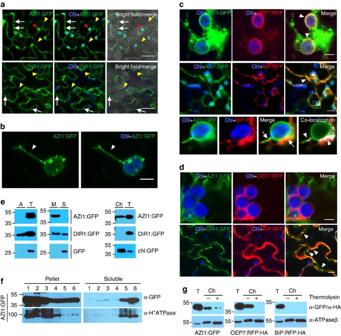Figure 1: Subcellular localization and membrane association properties of AZI1 and DIR1 in agrotransformedN. benthamiana. (a) Laser scanning confocal microscopy (confocal) micrographs showing localization of AZI1:GFP and DIR1:GFP controlled by Dex-inducible promoter in epidermal cells. White arrows: plasmodesmata-like structures/plasma membrane, yellow arrowheads: ER network/ER transcytoplasmic strands and red arrowheads: ring pattern surrounding chloroplasts. Scale bars, 30 μm. (b) ConfocalZ-series maximum intensity projection showing a close up view of AZI1:GFP surrounding chloroplasts and in stromule-like structures (white arrowheads). Scale bar, 5 μm. GFP, green; chloroplast autofluorescence, blue (Chl). (c,d) Confocal micrographs of AZI1:GFP (c) or DIR1:GFP (d) controlled by Dex-inducible promoter co-expressed with a chloroplast outer envelope protein marker (OEP7:RFP) or a ER marker (BiP:RFP) in epidermal cells. Bottom panels incare the close up of AZI1:GFP (from middle panels inset) in a stromule and surrounding a chloroplast showing contact sites with the ER marker (co-localization points are shown using a white mask on the merged image). Scale bars, 3 μm (upper panels) and 5 μm (middle panels). Arrowheads: co-localization. Arrows: contact sites between chloroplastic AZI1:GFP and BiP:RFP. Scale bar, 10 μm. GFP, green; RFP, red; chloroplast autofluorescence, blue (Chl). (e) Western blots of subcellular fractions: apoplast (A), microsomal (M), chloroplast (Ch), soluble (S) and total (T) fromN. benthamianaexpressing AZI1:GFP, DIR1:GFP, cytosolic GFP (GFP) or a GFP targeted to chloroplasts (chl:GFP). Bands were revealed using anti-GFP antibody. Similar results were observed in at least three independent experiments. (f) Membrane association strength of AZI1:GFP. Western blots, using the indicated antibodies, of pelleted and soluble proteins after total microsomal fraction treatments with: 1: control (150 mM NaCl); 2: 1.5 M NaCl; 3: 2 M urea; 4: 1% Triton; 5: 1% NP-40+0.5% deoxycolate; and 6: 1% SDS. H+ATPase is an integral membrane protein marker. (g) Thermolysin assay showing outer envelope membrane localization of AZI1:GFP. Intact chloroplasts were treated with control buffer (−) or thermolysin (+). Proteins from total homogenates (T) and chloroplast fractions (Ch) were revealed by western blots using the indicated antibodies. ATPaseβ is an internal chloroplast marker. Similar results were observed in two independent experiments. Figure 1: Subcellular localization and membrane association properties of AZI1 and DIR1 in agrotransformed N. benthamiana . ( a ) Laser scanning confocal microscopy (confocal) micrographs showing localization of AZI1:GFP and DIR1:GFP controlled by Dex-inducible promoter in epidermal cells. White arrows: plasmodesmata-like structures/plasma membrane, yellow arrowheads: ER network/ER transcytoplasmic strands and red arrowheads: ring pattern surrounding chloroplasts. Scale bars, 30 μm. ( b ) Confocal Z -series maximum intensity projection showing a close up view of AZI1:GFP surrounding chloroplasts and in stromule-like structures (white arrowheads). Scale bar, 5 μm. GFP, green; chloroplast autofluorescence, blue (Chl). ( c , d ) Confocal micrographs of AZI1:GFP ( c ) or DIR1:GFP ( d ) controlled by Dex-inducible promoter co-expressed with a chloroplast outer envelope protein marker (OEP7:RFP) or a ER marker (BiP:RFP) in epidermal cells. Bottom panels in c are the close up of AZI1:GFP (from middle panels inset) in a stromule and surrounding a chloroplast showing contact sites with the ER marker (co-localization points are shown using a white mask on the merged image). Scale bars, 3 μm (upper panels) and 5 μm (middle panels). Arrowheads: co-localization. Arrows: contact sites between chloroplastic AZI1:GFP and BiP:RFP. Scale bar, 10 μm. GFP, green; RFP, red; chloroplast autofluorescence, blue (Chl). ( e ) Western blots of subcellular fractions: apoplast (A), microsomal (M), chloroplast (Ch), soluble (S) and total (T) from N. benthamiana expressing AZI1:GFP, DIR1:GFP, cytosolic GFP (GFP) or a GFP targeted to chloroplasts (chl:GFP). Bands were revealed using anti-GFP antibody. Similar results were observed in at least three independent experiments. ( f ) Membrane association strength of AZI1:GFP. Western blots, using the indicated antibodies, of pelleted and soluble proteins after total microsomal fraction treatments with: 1: control (150 mM NaCl); 2: 1.5 M NaCl; 3: 2 M urea; 4: 1% Triton; 5: 1% NP-40+0.5% deoxycolate; and 6: 1% SDS. H + ATPase is an integral membrane protein marker. ( g ) Thermolysin assay showing outer envelope membrane localization of AZI1:GFP. Intact chloroplasts were treated with control buffer (−) or thermolysin (+). Proteins from total homogenates (T) and chloroplast fractions (Ch) were revealed by western blots using the indicated antibodies. ATPaseβ is an internal chloroplast marker. Similar results were observed in two independent experiments. Full size image Fractionation showed that DIR1:GFP was present in soluble, microsomal and apoplastic fractions ( Fig. 1e ), as previously reported [12] , [34] , [35] . AZI1:GFP was present in the microsomal and chloroplast fractions, but was not detected in soluble and apoplastic fractions ( Fig. 1e ). The controls, soluble GFP (GFP) and chloroplast-targeted GFP (chl:GFP), were found in soluble and chloroplastic fractions, respectively. The presence of AZI1:GFP in microsomal, but not soluble fractions prompted us to test the strength of association of AZI1:GFP with membranes. We treated the microsomal fraction with different salt concentrations, urea or detergents. Only treatments with NP40+deoxycolate or SDS completely solubilized the control integral membrane marker H + ATPase ( Fig. 1f ). These treatments also partially solubilized AZI1:GFP. Thus, AZI1:GFP has a strong association with membranes. After chloroplast purification, OEM proteins are susceptible to protease digestion [36] . In thermolysin-treated chloroplasts, AZI1:GFP was largely degraded indicating that at least the GFP portion was accessible to the cytosol, similar to OEP7 ( Fig. 1g ). In contrast, ATPaseβ, a protein that resides inside chloroplasts, was unaffected by thermolysin indicating that the isolated chloroplasts retained their integrity. Samples were not contaminated with ER, since BiP:RFP:HA was not present in the chloroplast fraction. Thus, DIR1 and AZI1 have overlapping, but also distinct cellular locations and biochemical properties, consistent with the proteins having different roles during SAR and AZA priming [10] . Chloroplast-localized AZI1 requires its PRR All AZI1 paralog members share hydrophobic N-termini annotated as signal peptides (SPs). However, AZI1 and some AZI1 paralogs also possess a PRR with distinctive lengths (AZI1, EARLI1, AZI3 to AZI6) or no PRR (AZI7) ( Fig. 2 ). In agrotransformed N. benthamiana , GFP fusions of AZI1 paralogs with long PRRs (EARLI1:GFP and AZI3:GFP) shared a similar localization pattern with AZI1:GFP, including prominent ring patterns surrounding chloroplasts and ER, whereas AZI5:GFP (short PRR) and AZI7:GFP lacked the chloroplast ring pattern ( Fig. 3a ). For EARLI1, fractionation confirmed that a pool of the protein localized to chloroplasts ( Supplementary Fig. 2 ). This shows a correlation between PRR length and chloroplast localization. GFP fusions to the N-termini of AZI1 and EARLI1, AZI3, AZI5 and AZI7 (lacking their C-terminal 8CM/LTP-like domains) recapitulated most of the patterns seen with full-length GFP fusion proteins ( Fig. 3b ). However, the perinuclear ER punctate/dense signals observed with full-length fusions ( Fig. 3a ) was missing with the N-terminal GFP fusion proteins ( Fig. 3b ). Thus, dense perinuclear localization was due to the 8CM domains of these proteins. To test whether a PRR is needed for the chloroplast OEM targeting, we localized a deletion version of AZI1:GFP lacking the PRR. AZI1ΔPRR:GFP showed no OEM chloroplast ring pattern signals, but did exhibit prominent ER and perinuclear ER signals ( Fig. 3c ). Thus, the PRR is needed for the chloroplast OEM targeting of AZI1 and probably also of its paralogs. 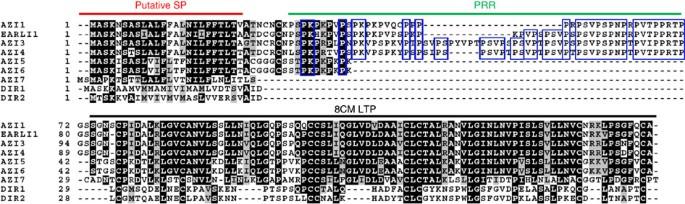Figure 2: ClustalW alignment ofArabidopsisAZI1 and DIR1 paralog proteins. The bars above the alignment indicates the putative signal sequence (SP), the N-terminal proline-rich region (PRR) and the lipid transfer protein eight cysteine motif (8CM–LTP). Black and grey boxes indicate identical or homologue sequences, respectively. Blue boxes indicate identical sequences along PRR. Figure 2: ClustalW alignment of Arabidopsis AZI1 and DIR1 paralog proteins. The bars above the alignment indicates the putative signal sequence (SP), the N-terminal proline-rich region (PRR) and the lipid transfer protein eight cysteine motif (8CM–LTP). Black and grey boxes indicate identical or homologue sequences, respectively. Blue boxes indicate identical sequences along PRR. 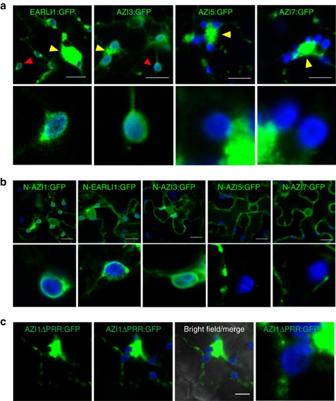Figure 3: AZI1’s paralog proteins subcellular localization in agrotransformedN. benthamiana. (a) Confocal micrographs showing localization of Dex-inducible EARLI1:GFP, AZI3:GFP, AZI5:GFP and AZI7:GFP. Yellow arrowheads: perinuclear ER punctate/dense signals and red arrowheads: ring pattern surrounding chloroplasts. Bottom panels: close up views of chloroplasts. (b) Confocal micrographs showing localization of Dex-inducible fusions to GFP with N-terminal regions of AZI1, EARLI1, AZI3, AZI5 and AZI7. Bottom panels: close up views of chloroplasts. (c) Confocal micrographs of AZI1 without its proline-rich region (AZI1ΔPRR:GFP). Right panel: close up views of chloroplasts. (a–c) Chloroplasts autofluorescence, blue; GFP, green. Scale bars, 15 μm. Full size image Figure 3: AZI1’s paralog proteins subcellular localization in agrotransformed N. benthamiana . ( a ) Confocal micrographs showing localization of Dex-inducible EARLI1:GFP, AZI3:GFP, AZI5:GFP and AZI7:GFP. Yellow arrowheads: perinuclear ER punctate/dense signals and red arrowheads: ring pattern surrounding chloroplasts. Bottom panels: close up views of chloroplasts. ( b ) Confocal micrographs showing localization of Dex-inducible fusions to GFP with N-terminal regions of AZI1, EARLI1, AZI3, AZI5 and AZI7. Bottom panels: close up views of chloroplasts. ( c ) Confocal micrographs of AZI1 without its proline-rich region (AZI1ΔPRR:GFP). Right panel: close up views of chloroplasts. ( a – c ) Chloroplasts autofluorescence, blue; GFP, green. Scale bars, 15 μm. Full size image AZI1 targeted to plastids increases during SAR induction In Arabidopsis , Dex-inducible AZI1:GFP complemented the SAR defect of azi1-1 Arabidopsis ( Supplementary Fig. 3a ), similar to constitutively expressed AZI1:GFP [32] . Upon Dex spray-treatment of two independent lines, AZI1:GFP showed similar localization as that seen in N. benthamiana . GFP signals, detected mainly in epidermal cells, co-localized with the autofluorescence of plastids ( Fig. 4a , Supplementary Fig. 3b ) and was observed in highly dynamic stromules ( Supplementary Movie 1 ). Z -series maximum intensity projections and three-dimensional reconstruction from optical sectioning showed AZI1:GFP in punctate/vesicle-like structures along ER transcytoplasmic strands and on chloroplast envelopes ( Fig. 4b , Supplementary Movie 2 ). AZI1:GFP was also observed in the PM ( Fig. 4b ). In addition, diffuse green fluorescence was also found within some nuclei ( Fig. 4b ; Supplementary Fig. 3b , Supplementary Movie 2 ). Because the signal was throughout the nucleus, the GFP signal was probably due to cleavage from the fusion protein. By using antibodies that specifically recognize AZI1 and EARLI1 (the most similar paralog of AZI1) monomers and SDS-resistant dimers in Arabidopsis [37] , we found that in wild-type (WT) Arabidopsis plants native AZI1/EARLI1 proteins are enriched similarly to ATPaseβ (chloroplastic marker) in the chloroplast fraction ( Fig. 4c ). As expected, BiP and FBP (ER and cytoplasm markers, respectively) are decreased in chloroplast fraction indicative of a low contamination in the fractionation ( Fig. 4c ). Interestingly, relative to a mock treatment, a SAR-inducing infection of Arabidopsis caused increased EARLI1/AZI1 in the chloroplast fraction, but did not affect total protein levels ( Fig. 4c , right graph). Together with localization data, this suggest that the plastid pool contributes to the systemic defence induction. 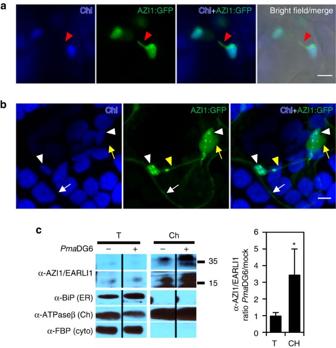Figure 4: Subcellular localization of AZI1 inArabidopsis. (a,b) Confocal micrographs of AZI1:GFP controlled by Dex-inducible promoter in transgenicArabidopsisseedlings showing AZI1 surrounding chloroplasts and in stromules and the ER. (b)Z-series maximum intensity projection showing localization of AZI1:GFP in epidermal cell chloroplasts. AZI1:GFP shows a punctate/vesicle-like localization along chloroplasts and an ER transcytoplasmic strand. White arrows: plasma membrane, white arrowheads: chloroplasts, yellow arrowheads: ER transcytoplasmic strand and red arrowheads: stromule. Yellow arrows: GFP fluorescence in a nucleus in close association to a chloroplast. Scale bar, 5 μm. GFP, green; chloroplast autofluorescence, blue (Chl). (c) Enrichment of AZI1–EARLI1 native proteins in chloroplast fraction after infection.ArabidopsisWT Col-0 leaves were mock-treated (−; 10 mM MgSO4) or infected with SAR-inducing strainPmaDG6 (+; OD600=0.0025). Extracts were prepared 21 h after inoculations. Proteins from total homogenates (T) and chloroplast fractions (Ch) were revealed by western blots using an anti-AZI1/EARLI1 polyclonal serum. Two bands are visualized corresponding to the native AZI1 and EARLI1 monomer and dimer sizes (∼17 and∼37 kD). BiP, ATPaseβ and FBP antibodies were used as ER, chloroplast and cytosolic markers, respectively. The same percentage of tissue mass (10% of input) was loaded for each fraction. Similar results were observed in three independent experiments. Right graph: AZI1–EARLI1 amount ratio between (−) and (+)PmaDG6. Levels are relative to the total protein content in each Coomassie blue-stained membrane lane as quantified by densitometry. The average with standard error from three biological replicates are shown. Asterisk indicate statistically significant differences as determined usingt-test (*P<0.05,n=3). Figure 4: Subcellular localization of AZI1 in Arabidopsis . ( a , b ) Confocal micrographs of AZI1:GFP controlled by Dex-inducible promoter in transgenic Arabidopsis seedlings showing AZI1 surrounding chloroplasts and in stromules and the ER. ( b ) Z -series maximum intensity projection showing localization of AZI1:GFP in epidermal cell chloroplasts. AZI1:GFP shows a punctate/vesicle-like localization along chloroplasts and an ER transcytoplasmic strand. White arrows: plasma membrane, white arrowheads: chloroplasts, yellow arrowheads: ER transcytoplasmic strand and red arrowheads: stromule. Yellow arrows: GFP fluorescence in a nucleus in close association to a chloroplast. Scale bar, 5 μm. GFP, green; chloroplast autofluorescence, blue (Chl). ( c ) Enrichment of AZI1–EARLI1 native proteins in chloroplast fraction after infection. Arabidopsis WT Col-0 leaves were mock-treated (−; 10 mM MgSO 4 ) or infected with SAR-inducing strain Pma DG6 (+; OD 600 =0.0025). Extracts were prepared 21 h after inoculations. Proteins from total homogenates (T) and chloroplast fractions (Ch) were revealed by western blots using an anti-AZI1/EARLI1 polyclonal serum. Two bands are visualized corresponding to the native AZI1 and EARLI1 monomer and dimer sizes ( ∼ 17 and ∼ 37 kD). BiP, ATPaseβ and FBP antibodies were used as ER, chloroplast and cytosolic markers, respectively. The same percentage of tissue mass (10% of input) was loaded for each fraction. Similar results were observed in three independent experiments. Right graph: AZI1–EARLI1 amount ratio between (−) and (+) Pma DG6. Levels are relative to the total protein content in each Coomassie blue-stained membrane lane as quantified by densitometry. The average with standard error from three biological replicates are shown. Asterisk indicate statistically significant differences as determined using t -test (* P <0.05, n =3). Full size image Arabidopsis EARLI1 is required for SAR and AZA priming Since AZI1 and EARLI1 both have roles in stress tolerance [37] , [38] , we tested if they function similarly in pathogen defence. A SAR-inducing strain ( Pma DG6) grew to the same extent in earli1-1 and WT ( Supplementary Fig. 4a ). Moreover, similar to azi1-1 , earli1-1 loss of function plants did not show SAR or AZA-conferred systemic resistance to virulent Pseudomonas syringae ( Fig. 5a,b ). Both azi1-1 and earli1-1 showed slower induction of pathogenesis-related protein 1 (PR1) than WT after secondary infection ( Fig. 5c,d ) indicating they have priming defects. The earli1-1 plants were not generally hypersusceptible to P. syringae , since the mock-treated controls of earli1-1 and WT showed similar pathogen growth ( Fig. 5a,b ). Thus, EARLI1, the closest AZI1 paralog, is a SAR/AZA-priming component. 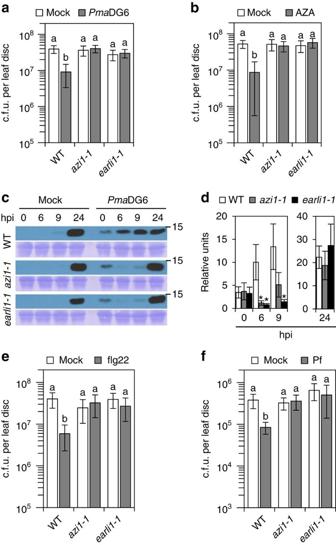Figure 5: Induction of systemic defence inArabidopsis azi1andearli1mutants. (a,b,e,f) Growth of the virulent bacteriaPmaDG3 on WT Col-0,azi1-1andearli1-1plants 3 days post infection (OD600=0.0001).PmaDG3 was infiltrated in distal upper leaves after 2 days of lower leaf treatment with mock (10 mM MgSO4) or strainPmaDG6 (OD600=0.01) to test SAR (a), control MES (mock) or AZA to test AZA-conferred systemic immunity (b), water (mock) or 100 nM flg22 to test mSAR (e); or after 3 weeks of mock (10 mM MgSO4) orPfstrain root inoculation to test ISR (f). The average of c.f.u. per leaf disc plus/minus 95% confidence interval from foura, three (b,e) and two (f) independent experiments (each one with eight biological replicates) is shown. Graphyaxes are in log10 scale. (c) PR1 protein levels in total extracts in WT Col-0 andazi1-1andearli1-1plants at different times post infiltration ofPmaDG3 (OD600=0.01) to test PR1 priming in plants previously mock-treated orPmaDG6-treated to induce SAR (as ina). The blots stained with Coomassie blue are presented to show loading. Similar results were observed in four independent experiments. (d) Quantification of PR1 levels in (c)PmaDG6 samples relative to the total protein content in each CBB membrane lane as quantified by densitometry. The average with standard error from four independent experiments are shown. Ina,b,e,fdifferent letters indicate statistically significant differences (P<0.01, analysis of variance (ANOVA), SNK test). Graphyaxes are in log10 scale. Ind, the asterisk indicates statistically significant differences versus WT at each time point determined usingt-test (*P<0.05,n=4). In (c) and (d) hpi indicates hours post-infection. Figure 5: Induction of systemic defence in Arabidopsis azi1 and earli1 mutants. ( a , b , e , f ) Growth of the virulent bacteria Pma DG3 on WT Col-0, azi1-1 and earli1-1 plants 3 days post infection (OD 600 =0.0001). Pma DG3 was infiltrated in distal upper leaves after 2 days of lower leaf treatment with mock (10 mM MgSO 4 ) or strain Pma DG6 (OD 600 =0.01) to test SAR ( a ), control MES (mock) or AZA to test AZA-conferred systemic immunity ( b ), water (mock) or 100 nM flg22 to test mSAR ( e ); or after 3 weeks of mock (10 mM MgSO 4 ) or Pf strain root inoculation to test ISR ( f ). The average of c.f.u. per leaf disc plus/minus 95% confidence interval from four a , three ( b , e ) and two ( f ) independent experiments (each one with eight biological replicates) is shown. Graph y axes are in log10 scale. ( c ) PR1 protein levels in total extracts in WT Col-0 and azi1-1 and earli1-1 plants at different times post infiltration of Pma DG3 (OD 600 =0.01) to test PR1 priming in plants previously mock-treated or Pma DG6-treated to induce SAR (as in a ). The blots stained with Coomassie blue are presented to show loading. Similar results were observed in four independent experiments. ( d ) Quantification of PR1 levels in ( c ) Pma DG6 samples relative to the total protein content in each CBB membrane lane as quantified by densitometry. The average with standard error from four independent experiments are shown. In a , b , e , f different letters indicate statistically significant differences ( P <0.01, analysis of variance (ANOVA), SNK test). Graph y axes are in log10 scale. In d , the asterisk indicates statistically significant differences versus WT at each time point determined using t -test (* P <0.05, n =4). In ( c ) and ( d ) hpi indicates hours post-infection. Full size image AZI1 and EARLI1 are required for mSAR and ISR in Arabidopsis AZI1 and EARLI1 (as well as AZI3/4 ) are induced by MAMPs and expressed in roots (genevestigator [39] ). Local callose induction by the MAMP flg22 was similar in azi1-1 , earli1-1 and WT ( Supplementary Fig. 4b ). However, we found that both AZI1 and EARLI1 are needed for systemic resistance induced by flg22 [7] ( Fig. 5e ). We also tested the role of AZI1 and EARLI1 in ISR triggered by root-colonizing P. fluorescens WCS417r [8] . After inoculation of roots with P. fluorecens , only WT, but not azi1-1 or earli1-1 , showed a significant reduction of P. syringae growth in distal-infected leaves ( Fig. 5f ). This indicates that AZI1 and EARLI1 are needed for mSAR and ISR. SAR complexes include LTP and LTP-like proteins AZI1 can form a complex with DIR1 [32] . To test whether EARLI1 might also form complexes, we co-expressed pairwise combinations of EARLI1, AZI1 and DIR1 in N. benthamiana . We detected complexes that contained each pair of proteins tested, as measured by co-immunoprecipitation (co-IP) ( Fig. 6a ). The presence of highly dithiothreitol-resistant dimers/tetramers in the blots ( Supplementary Fig. 5 ) supports the idea that these 8CM proteins form SAR complexes. Furthermore, DIR1:RFP co-localized with AZI1:GFP and EARLI1:GFP at perinuclear ER and plasmodesmata ( Fig. 6b ), as previously reported for AZI1/DIR1 [32] . We also detected co-localization at sites that abut chloroplasts, which are likely chloroplast–ER contact sites ( Fig. 6c ) and possible stromule–ER contact sites ( Fig. 6d ). As expected, no co-immunoprecipitation or co-localization was found between control soluble GFP and DIR1:RFP ( Fig. 6a , Supplementary Fig. 6 ). Thus, 8CM-containing complexes may connect organelles and structures in cells, which may be important for transmission of systemic signals. 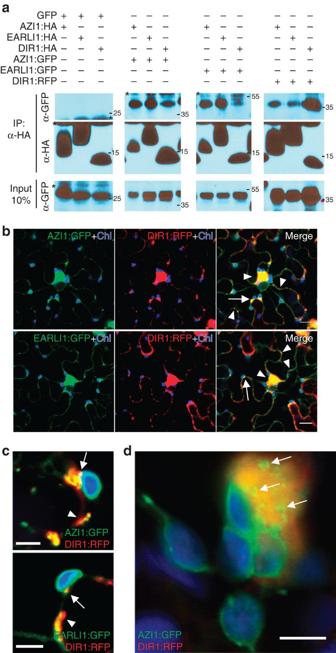Figure 6: AZI1, EARLI1 and DIR1 complexes and co-localization in agrotransformedN. benthamiana. (a) Co-immunoprecipitation of AZI1, EARLI1 and DIR1. AgrotransformedN. benthamianatissues co-expressing combinations of control GFP (GFP), AZI1:GFP/:HA, EARLI1:GFP/:HA or DIR1:RFP/:HA were used. Complexes were immunoprecipitated with HA antibody. IP: immunoprecipitation. Both input (bottom panels) and IP (upper panels) protein samples were analysed by western blot using the indicated antibodies. Similar results were observed in three (between AZI1/DIR1 combinations) and two (between AZI1/EARLI1/DIR1 combinations) independent experiments. Asterisks indicate unspecific bands. (b,c) Confocal micrographs showing localization of co-expressed AZI1:GFP or EARLI1:GFP and DIR1:RFP inN. benthamianaepidermal cells. (c) Close up view of AZI1:GFP or EARLI1-GFP and DIR1:RFP co-localization at ER and chloroplast–ER contact sites. (d)Z-series maximum intensity projection showing close up view of AZI1:GFP and DIR1:RFP co-localization in chloroplast–ER and stromule–ER contact sites. Arrowheads: co-localization at ER, perinuclear ER and plasmodesmata; arrows: co-localization at chloroplast/stromule–ER contact sites. The micrographs show GFP, green; RFP, red; chloroplasts autofluorescence, blue (Chl). The yellow/orange colour in the merged images indicates co-localization. Scale bars, 15 μm (b) and 5 μm (c,d). Figure 6: AZI1, EARLI1 and DIR1 complexes and co-localization in agrotransformed N. benthamiana . ( a ) Co-immunoprecipitation of AZI1, EARLI1 and DIR1. Agrotransformed N. benthamiana tissues co-expressing combinations of control GFP (GFP), AZI1:GFP/:HA, EARLI1:GFP/:HA or DIR1:RFP/:HA were used. Complexes were immunoprecipitated with HA antibody. IP: immunoprecipitation. Both input (bottom panels) and IP (upper panels) protein samples were analysed by western blot using the indicated antibodies. Similar results were observed in three (between AZI1/DIR1 combinations) and two (between AZI1/EARLI1/DIR1 combinations) independent experiments. Asterisks indicate unspecific bands. ( b , c ) Confocal micrographs showing localization of co-expressed AZI1:GFP or EARLI1:GFP and DIR1:RFP in N. benthamiana epidermal cells. ( c ) Close up view of AZI1:GFP or EARLI1-GFP and DIR1:RFP co-localization at ER and chloroplast–ER contact sites. ( d ) Z -series maximum intensity projection showing close up view of AZI1:GFP and DIR1:RFP co-localization in chloroplast–ER and stromule–ER contact sites. Arrowheads: co-localization at ER, perinuclear ER and plasmodesmata; arrows: co-localization at chloroplast/stromule–ER contact sites. The micrographs show GFP, green; RFP, red; chloroplasts autofluorescence, blue (Chl). The yellow/orange colour in the merged images indicates co-localization. Scale bars, 15 μm ( b ) and 5 μm ( c , d ). Full size image AZI1 and EARLI1 are needed locally for SAR establishment SAR components might act at one or more steps: during initial immunization, later in distal tissue to establish a primed state and/or during SAR manifestation. We used a Dex painting method to drive local inducible AZI1:HA or EARLI1:HA expression in azi1-1 plants only after Dex treatment ( Fig. 7a , right panels). When AZI1 or EARLI1 were expressed only at the local site treated with SAR-inducing Pma DG6 bacteria, SAR was restored, as evidenced by reduced P. syringae growth in distal leaves ( Fig. 7a ). As expected, WT control plants showed normal SAR with or without Dex treatment. The results suggest that AZI1 and EARLI1 function similarly. That is, they are needed at a critical threshold level at the local immunization site. 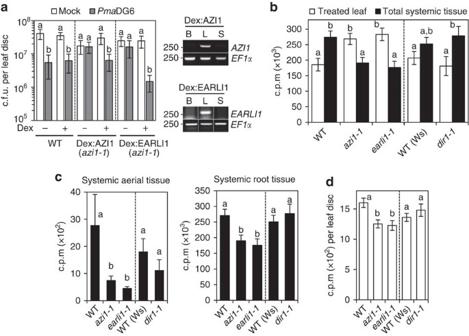Figure 7: Functional roles of AZI1 and EARLI1 in SAR and AZA movement. (a) Rescue ofazi1-1SAR-defective phenotype by locally induced AZI1 or EARLI1. Three lower leaves of Dex:AZI1:HA/azi1-1and Dex:EARLI1:HA/azi1-1were brushed with 3 μM Dex to locally induce AZI1/EARLI1, and 21 h later immunized by infiltration with 10 mM MgSO4(mock) orPmaDG6 (DG6). To test SAR, distal leaves were infected withPmaDG3 2 days later. The average of c.f.u. per leaf disc ±95% confidence interval from four (WT and Dex:AZI1) and three (Dex:EARLI1) independent experiments (each with eight biological replicates) is shown. Different letters indicate significant differences between treatments in WT, Dex:AZI1 and Dex:EARLI1 (P<0.01, analysis of variance (ANOVA), SNK test).yAxes show log10 scale. Right panels: RT–PCR ofAZI1andEARLI1transcripts. Leaves were collected (treated, L; distal, S) 21 h after brushing L with 3 μM Dex; B indicates basal (untreated) expression control. Expression ofEF1α was used as an internal standard. (b–d) Movement and uptake of [14C]azelaic acid (14C-AZA) in WT (Col-0, Ws) or mutants (azi1-1,earli1-1anddir1-1). (b)In planta14C-AZA movement. Quantification of radioactivity remaining 24 h after application of14C-AZA in treated leaf, white bar, and the estimated radiolabel in total systemic tissues (c.p.m. initially applied minus c.p.m. remaining in the treated leaf), black bar. (c) Quantification of radioactivity in systemic aerial tissues (without treated leaf) 24 h after application of14C-AZA in the same plants asb, and estimation of radioactivity in roots (total systemic tissues estimated c.p.m. inbminus c.p.m. quantified in aerial tissues). (b,c) Graphs represent the average with standard error from five independent experiments for WT andazi1-1(n=18) and three independent experiments forearli1-1, Ws anddir1-1(n=10). (d)14C-AZA uptake. Quantification of radioactivity in leaf discs after floating on14C-AZA for 3 h followed by three washes during 1 h. The average with standard error from two independent experiments (n=30) is shown. Inb–d, different letters indicate statistically significant differences between WT Col,azi1-1,earli1-1and WT Ws,dir1-1(P<0.01, ANOVA, SNK test). Figure 7: Functional roles of AZI1 and EARLI1 in SAR and AZA movement. ( a ) Rescue of azi1-1 SAR-defective phenotype by locally induced AZI1 or EARLI1. Three lower leaves of Dex:AZI1:HA/ azi1-1 and Dex:EARLI1:HA/ azi1-1 were brushed with 3 μM Dex to locally induce AZI1/EARLI1, and 21 h later immunized by infiltration with 10 mM MgSO 4 (mock) or Pma DG6 (DG6). To test SAR, distal leaves were infected with Pma DG3 2 days later. The average of c.f.u. per leaf disc ±95% confidence interval from four (WT and Dex:AZI1) and three (Dex:EARLI1) independent experiments (each with eight biological replicates) is shown. Different letters indicate significant differences between treatments in WT, Dex:AZI1 and Dex:EARLI1 ( P <0.01, analysis of variance (ANOVA), SNK test). y Axes show log10 scale. Right panels: RT–PCR of AZI1 and EARLI1 transcripts. Leaves were collected (treated, L; distal, S) 21 h after brushing L with 3 μM Dex; B indicates basal (untreated) expression control. Expression of EF1 α was used as an internal standard. ( b – d ) Movement and uptake of [ 14 C]azelaic acid ( 14 C-AZA) in WT (Col-0, Ws) or mutants ( azi1-1 , earli1-1 and dir1-1 ). ( b ) In planta 14 C-AZA movement. Quantification of radioactivity remaining 24 h after application of 14 C-AZA in treated leaf, white bar, and the estimated radiolabel in total systemic tissues (c.p.m. initially applied minus c.p.m. remaining in the treated leaf), black bar. ( c ) Quantification of radioactivity in systemic aerial tissues (without treated leaf) 24 h after application of 14 C-AZA in the same plants as b , and estimation of radioactivity in roots (total systemic tissues estimated c.p.m. in b minus c.p.m. quantified in aerial tissues). ( b , c ) Graphs represent the average with standard error from five independent experiments for WT and azi1-1 ( n =18) and three independent experiments for earli1-1 , Ws and dir1-1 ( n =10). ( d ) 14 C-AZA uptake. Quantification of radioactivity in leaf discs after floating on 14 C-AZA for 3 h followed by three washes during 1 h. The average with standard error from two independent experiments ( n =30) is shown. In b – d , different letters indicate statistically significant differences between WT Col, azi1-1 , earli1-1 and WT Ws, dir1-1 ( P <0.01, ANOVA, SNK test). Full size image AZI1 and EARLI1 are needed for AZA uptake and movement The 8CM-domain proteins AZI1, EARLI1 and/or DIR1 are candidates for transporting or acting in the perception of AZA, which resembles a small lipid. Isotopically labelled AZA is mobile in Arabidopsis , with a portion of heavy isotope- and/or radio-labelled AZA remaining intact and a portion becoming modified [10] , [32] . We applied 14 C-AZA [40] to different mutants and monitored the distribution of label in whole plants or the uptake into leaf discs. Movement of label from one leaf (the application site) to total systemic tissues (aerial stem/leaves and roots) was significantly reduced in azi1-1 and earli1-1 compared to Col WT plants ( Fig. 7b,c ). In WT, a large amount of the signal that moved to aerial tissues was detected in very young leaves ( Supplementary Fig. 7 ). Interestingly, based on the amount of label that exited the treated leaf and was mobilized to aerial tissue ( Fig. 7b,c ), we estimated that a lot of signal moved systemically to the roots. In contrast, AZA systemic movement was not reduced in dir1-1 compared with Wassilewskija (Ws) WT parent plants ( Fig. 7b,c ). Both azi1-1 and earli1-1 but not dir1 showed significant decreases in label uptake into leaf discs ( ∼ 25%) compared to WT ( Fig. 7d ). Label uptake was the same in dir1-1 and WT WS leaf discs. Systemic movement or uptake in leaf discs of 14 C-sucrose was not different between any mutants and the respective WT plants ( Supplementary Fig. 8a–c ) indicating that these mutations are not affecting the general phloematic fluxes. Yu et al . [32] reported that azi1 did not differ from WT in 14 C-AZA movement. However, accounting for the total pool of label applied to plants was not done previously. In addition, here AZA was applied in a small drop instead of infiltrated using a large volume of liquid, which may affect how much AZA can be uploaded to reach the vasculature. These data show that movement and uptake of AZA (and possibly AZA derivatives) partially depends on AZI1 and EARLI1, but not DIR1. AZI1 subcellular dynamics To gain insight into how AZI1 could be functioning, we analysed its dynamics inside cells. Live cell imaging of N. benthamiana showed that AZI1:GFP was present in vesicle-like structures that moved rapidly to and from chloroplasts to the cytoplasm ( Fig. 8a ). These vesicle-like structures moved in close association with ER transcytoplasmic strands connecting chloroplasts, ER and the PM ( Supplementary Movie 3 ). Moreover, using the AZI1 N-terminal GFP fusion, we observed the movement of a chloroplast attached to the ER network through a stromule (chloroplast/ER contact site) structure where N-AZI1:GFP was localized ( Fig. 8b and Supplementary Movie 4 ). In contrast, DIR1:GFP showed dynamic movement, but mainly in the ER ( Supplementary Movie 5 ). 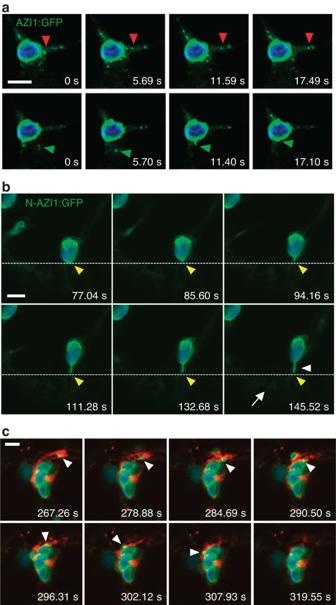Figure 8: Dynamics of AZI1 in chloroplasts outer envelope by live imaging confocal microscopy in agrotransformedN. benthamiana. (a) Time series micrographs showing dynamic localization of AZI1:GFP controlled by Dex-inducible promoter in vesicle-like structures moving in (green arrowheads) and out (red arrowheads) from chloroplasts. (b) Time series micrographs showing dynamic localization of N-terminal sequence GFP fusion proteins of AZI1 controlled by Dex-inducible promoter in chloroplast, stromule and ER network connections. White arrowhead: stromule-localized AZI1:GFP, white arrow: ER-localized AZI1:GFP and yellow arrowheads: chloroplast/ER contact site. (c) Time series micrographs showing dynamic localization of N-terminal sequence GFP fusion proteins of AZI1 and BiP:RFP in chloroplasts and ER network connections. White arrowheads: dynamic chloroplast/ER contact sites. Scale bars, 5 μm (a–c). Chloroplast autofluorescence, blue; GFP, green; RFP, red. Figure 8: Dynamics of AZI1 in chloroplasts outer envelope by live imaging confocal microscopy in agrotransformed N. benthamiana . ( a ) Time series micrographs showing dynamic localization of AZI1:GFP controlled by Dex-inducible promoter in vesicle-like structures moving in (green arrowheads) and out (red arrowheads) from chloroplasts. ( b ) Time series micrographs showing dynamic localization of N-terminal sequence GFP fusion proteins of AZI1 controlled by Dex-inducible promoter in chloroplast, stromule and ER network connections. White arrowhead: stromule-localized AZI1:GFP, white arrow: ER-localized AZI1:GFP and yellow arrowheads: chloroplast/ER contact site. ( c ) Time series micrographs showing dynamic localization of N-terminal sequence GFP fusion proteins of AZI1 and BiP:RFP in chloroplasts and ER network connections. White arrowheads: dynamic chloroplast/ER contact sites. Scale bars, 5 μm ( a – c ). Chloroplast autofluorescence, blue; GFP, green; RFP, red. Full size image To study the dynamics of AZI1/ER contact sites in more detail, we co-expressed an N-terminal AZI1:GFP fusion and the ER marker BiP:RFP. Interestingly, we found highly dynamic co-localized signals, particularly between the chloroplast-located AZI1:GFP and BiP:RFP ( Fig. 8c ; Supplementary Movie 6 , Supplementary Movie 7 ). The pattern of movement of AZI1 and the AZI1/ER contact sites together with its regulation by infection ( Fig. 4c ) is consistent with AZI1 complexes facilitating transport of SAR signals, and connecting chloroplast envelope membranes to different organelles and/or subcellular structures. SAR protects plants over an extended period and involves an energy-saving priming of the defences in systemic (distal) tissues after a first infection. We showed here that the AZI1 paralog EARLI1 is a new SAR component and that along with AZI1, it is also essential for AZA-conferred systemic resistance, mSAR and ISR. Thus, these HyPRPs are part of a central mechanism used for systemic disease resistance programs. Both AZI1 and EARLI1 are needed for AZA movement to distal tissues. AZI1 and EARLI1 are membrane proteins localized in the PM, ER and, interestingly, chloroplast outer envelopes. Production of SAR signals, including AZA, occurs in chloroplasts [22] , [41] . Therefore, we propose that a central function of AZI1/EARLI1, which are needed at the immunization site, is to facilitate mobilization of SAR signals from where they are made (chloroplasts) to vasculature uploading sites (ER–plasmodesmata and PM/apoplast). Given their requirement for efficient AZA mobilization, they likely also have key roles in the movement of AZA during establishment of SAR, mSAR and ISR. DIR1’s role may be more closely related to signal perception [10] . Remarkably, chloroplast targeting of AZI1 (and some AZI1 paralogs) employs an N-terminal bipartite signal that to our knowledge was not described before in plants. In Arabidopsis seedlings, AZA can move from local to distal aerial tissues [10] . In adult plants, AZA and AZA derivatives are also mobile [32] . Interestingly, AZA can also move from one leaf to roots. This raises the possibility that AZA priming may have a role in underground tissues. In support of this idea, foliar pathogens can trigger disease resistance in roots [42] . Future studies on this aspect is of major interest to know if/how aerial infection can influence root defences or even shape the normal root-associated microbiota. AZI1 and EARLI1 are needed for normal movement of AZA (or AZA-derived molecule(s)). Although AZA resembles a small lipid, it is probable that the size/structure of AZA will not allow a direct binding to AZI1/EARLI1’s 8CM–LTP motif [30] . Since AZA may be esterified to a lipid until its release by a lipase [22] , [43] , AZI1/EARLI1 may bind an AZA-carrying lipid(s). Thus, AZI1/EARLI1 may facilitate AZA movement by binding a lipid–AZA, such as the polar lipidic AZA derivatives found in plants after AZA treatment [32] . Chloroplasts play key roles in plant defence against biotic stresses [44] , [45] . This appears to be especially true during systemic defence programs, where among the proposed SAR signals, several are directly related to chloroplast metabolism [10] , [12] , [15] , [16] , [17] . Indeed, AZA is generated in plastid membranes [22] . Moreover, during SAR-inducing infections AZA levels increase [10] , [12] , [32] , probably due to an increase of nitric oxide/reactive oxygen species in chloroplasts [31] , [46] . AZI1, EARLI1 and AZI3 are upregulated by AZA and/or conditions that promote non-enzymatic lipid peroxidation [47] . Thus, the regulation and chloroplast OEM location of these HyPRPs during infection is consistent with them having roles in AZA mobilization. MCSs between ER/chloroplast and stromules/ER (or transcytoplasmic ER strands) are major places were lipid exchange occurs [26] , [27] , [28] . These MCSs are typically enriched in LTPs that tether opposite membranes by protein–protein/protein–lipid interactions [24] , [25] . The localization of AZI1 and EARLI1 and enrichment of AZI1 at dynamic contact sites indicates that AZI1/EARLI1 may function to facilitate AZA or lipid–AZA movement. Moreover, MCSs not only assist in lipid exchange, but also ensure and provide specificity [29] . This could explain why DIR1, an AZI1/EARLI1 interactor and possible member of a ‘SAR complex’, could be transporting lipidic signals other than AZA [17] , [32] . AZI1, EARLI1 and AZI3–7 paralogs belong to the HyPRP family proteins that were hypothesized to be associated with the cell wall due to the abundance of prolines in the PRR [30] , [48] . However, the PRR is needed for chloroplast OEM localization in AZI1. Therefore, the role of the PRR in other HyPRPs outside the AZI1 family may be similar. Many chloroplast OEM proteins use a signal anchor mechanism to target plastids, which requires a transmembrane domain usually annotated as a SP of a certain hydrophobicity [33] . These proteins were not described as having a PRR and therefore there might be distinct mechanisms for targeting the AZI1 family and perhaps other HyPRPs, possibly due to a requirement for them in multiple subcellular sites. AZI1 family proteins possess N-terminal bipartite ‘signals’ (putative SP+PRR) with different lengths of PRRs that drive dynamic localization between plastid OEMs, ER and/or the PM. These proteins appear to use a targeting mechanism that involves the ER/secretory pathway. Carbonic anhydrase 1 (CAH1) is one of the very few higher plant proteins also known to target chloroplast through the endomembrane system [49] . However, CAH1 localizes to the stroma indicating its targeting mechanism must be different from AZI1, at least in part. Interestingly, Apicomplexa organisms use N-terminal bipartite signals for plastid (apicoplast)-targeted proteins [50] . Apicoplast targeting signals are characterized by a plastid transit peptide next to the SP. An algorithm developed to predict apicoplast targeting proteins based on the SP and an adjacent transit peptide (the PATs program [51] ) correctly predicts the plastid localizations of AZI1 family members and CAH1. How this targeting system works at the molecular level in higher plants will be an interesting topic for future work. AZI1 and EARLI1 are key factors in SAR-priming establishment, needed specifically at the site of the first immunization, possibly by affecting AZA or lipid–AZA mobilization from local leaves to distal sites. An interesting finding is that AZI1:GFP that complements azi1-1 is mainly detected in epidermal cells. We speculate that these cells are a significant place for AZI1 function. Pavement cells are the first contact point for interaction with the environment and microbes. Importantly, their plastids are specialized organelles in which fatty acids and cuticle components destined for the epidermal cell surface are synthesized [52] . The fact that fatty acids are the precursors of AZA and other oxylipins [41] and an intact cuticle is needed for SAR [13] supports the idea that epidermal cells may be important for long-distance defence signalling. AZI1 and EARLI1 represent novel shared components between ISR and SAR. Because AZA and other oxylipins (or lipid–oxylipins) can be also generated in roots [41] , [53] , it is possible that AZI1/EARLI1 could facilitate trafficking of these types of signals from roots to aerial tissue. Interestingly, AZI1 is induced in roots after ISR-inducing bacteria colonization [54] . A common feature of different stress signalling pathways may be the remodelling of chloroplast OEM lipids as well as PM lipids and reactive oxygen species production [55] , [56] . Moreover, several HyPRPs from different plant species have been reported to have roles in abiotic stress tolerance [38] , [57] , [58] , [59] . Thus, it is also possible that all AZI1 family members (and maybe other HyPRP proteins) may be adapted to promote lipid-based signalling during defence induction under diverse stresses. Plants and vectors All plants were 25- to 28-day-old Arabidopsis thaliana in the Columbia-0 (Col-0) or WS background, except where indicated. azi1-1 , earli1-1 (Col-0 background) and dir1-1 (WS background) were previously described [10] , [11] , [58] . Plants were grown under 12-h day (08:00 to 20:00) and 12-h night conditions at 20 °C, 200–230 μmol s −1 m −2 light at rosette level and 50–70% relative humidity [10] . N. benthamiana were grown at 24 °C and with 16-h day light. Plants were grown for 4 weeks before Agrobacterium tumefaciens -mediated transient transformation. All vectors and primers used in this study are listed in Supplementary Table 1 . The full coding region of Arabidopsis AZI1, EARLI1, AZI3, AZI5, AZI7 and DIR1 and the N-terminal region of AZI1, EARLI1, AZI3, AZI5 and AZI7 (SP+PRR) were amplified with PCR primers linked to specific sequences compatible with the GATEWAY cloning procedure, and introduced into the plant expression vector pBAV150(ref. 60 ). Full-length coding region of AZI1, EARLI1 and DIR1 were also introduced in pBAV154 (ref. 60 ). In addition, AZI1 was cloned into pSITEII-7N1 expression vector (CD3-1646/ABRC [61] ). To generate the Δ 32–76 AZI1 (AZI1ΔPRR) proper fragments were linked by PCR creating the deletion and then introduced into pBAV150. The chloroplast outer envelope protein marker OEP7 (OEP7:RFP) and the ER marker BiP (BiP:RFP) fused to RFP were amplified by PCR from pUC-OEP7:RFP and pUC-BiP:RFP vectors, kindly provided by Dr Inhwan Hwang [33] , and introduced in pBAV154. All the resulting plasmids allowed the expression of the transgenes with C-terminal GFP (pBAV150) or HA epitope tag (pBAV154) controlled by the Dex-inducible promoter. pSITEII-7N1 vector allowed the expression of AZI1 with C-terminal GFP (Dendra2) driven by the constitutive 35S promoter. The vector allowing DIR1 expression fused to C-terminal RFP (pSITE-DIR1:RFP) under constitutive promotor 35S, was a gift from Dr Pradeep Kachroo [12] . The plastid-targeted GFP (chl:GFP) was obtained from ABRC (pt-gk/CD3-995/ABRC [61] ). Transgenic plants were established by dipping azi1-1 mutant flowers into suspensions of A. tumefaciens GV3101 strain harbouring the pBAV150:AZI1, pBAV154:AZI1 and pBAV154:EARLI1 [62] , and then selected on Murashige and Skoog media (Sigma-Aldrich) supplemented with Basta (10 μg ml − 1 ). F 3 or F 4 generation plants were used for experiments. Systemic resistance assays To evaluate systemic resistance, distal leaves were syringe-inoculated with virulent P. syringae pv. maculicola ES4326 carrying an empty vector ( Pma DG3; optical density at a wavelength of 600 nm, OD 600 =0.0001) [63] two days after SAR, mSAR or 3 weeks after ISR induction. Growth was quantified using eight leaves from different plants 3 days after Pma DG3 inoculation. For SAR induction, three lower leaves were infiltrated with P. syringae pv. maculicola ES4326 strain carrying AvrRpt2 ( Pma DG6; OD 600 =0.01) [63] . For mSAR, three lower leaves were infiltrated with 100 nM flg22. ISR was induced by transplanting 12-day-old sand-grown seedlings into a soil/sand mixture (12:5) inoculated with P. fluorescens WCS417r to a final density of 5 × 10 7 c.f.u. g − 1 soil (mixed thoroughly with 10 9 c.f.u. ml − 1 suspension) [8] . To analyse priming of PR1 induction, distal leaves from mock- or SAR-induced plants were syringe-inoculated with Pma DG3 (OD 600 =0.01) and protein samples were obtained at different times post infection. At least three leaves from three different plants were used per time point. To analyse the local rescue of azi1-1 mutation by AZI1 or EARLI1, three lower leaves of transgenic Arabidopsis azi1-1 plants carrying pBAV154:AZI1 or pBAV154:EARLI1 constructs were gently painted (with a ¼″ Angler Shader paintbrush, Princeton Art and Brush Co.) with 3 μM Dex plus 0.1% Tween 20 solution 21 h before inoculation of the same leaves with Pma DG6 used to trigger SAR. To show AZI1:GFP functionality in Arabidopsis transgenic azi1-1 plants carrying pBAV150:AZI1 construct were sprayed with 30 μM Dex plus 0.1% Tween 20 solution 21 h before analysing SAR induction. Exogenous application of AZA AZA (C 9 H 16 O 4 , molecular weight 188.22, Sigma-Aldrich) was dissolved in 5 mM 2-[ N -morpholino]ethanesulfonic acid (MES, pH 5.6; Sigma-Aldrich) to increase its solubility and stabilize pH. Solutions of 1 mM AZA or only MES (mock control) were directly infiltrated into three lower leaves with a needleless syringe 2 days before Pma DG3 inoculation in systemic leaves [10] . 14 C-AZA movement and uptake assays For movement and uptake assays, 14 C-AZA [40] was used. For in planta movement, 14 C-AZA stock solution (specific activity 16 mCi mmol −1 ) was evaporated to complete dryness under a stream of nitrogen gas (to remove the acetonitrile and formic acid solvent). The dried precipitate was dissolved to concentration of 0.5 μCi per 20 μl of 5 mM MES (pH 5.6) containing 0.1% Triton X-100 detergent. 14 C-AZA was applied as a 20 μl drop to the abaxial side of a fully expanded Arabidopsis leaf (0.5 μCi per plant; covering ∼ 3–5 mm 2 of the leaf area). Plants were covered for 24 h to maintain humidity and then quantified as follows: the treated leaf and the rest of the aerial tissue were dried separately, cut in small pieces, placed in scintillation vials and dissolved in scintillation cocktail for radioactivity quantification. To calculate the estimated amount of label moved to root and total systemic tissues, we consider the initial c.p.m. applied. Radioactivity (c.p.m.) was quantified in a liquid scintillation counter (LS 6000 IC, Beckman). c.p.m. in the initial drop applied (4.6 × 10 5 c.p.m.) was determined by averaging measurements from three leaves that were drop-treated with 14 C-AZA and immediately dried. For 14 C-sucrose movement control 0.5 μCi (sucrose [ 14 C(U)], 435 mCi mmol − 1 , Perkin Elmer) was also used. 14 C-sucrose radioactivity in the initial drop applied was 5.9 × 10 5 c.p.m.. For uptake assays 15 leaf discs (4 mm diameter) from 8–9 plants were collected per replicate, incubated in 15.5 μM 14 C-AZA/1 mM cold AZA solution (0.744 × 10 − 3 μCi in 3 ml bathing medium; 5 mM MES; pH 5.6) for 3 h in a six-well plate, washed three times with only 5 mM MES (pH 5.6) for a total of 1 h, dried and dissolved in scintillation cocktail. For uptake control 14 C-sucrose was used [64] . mRNA analysis Total RNA isolation and reverse transcription were done using Trizol reagent and Masterscript RT–PCR system, respectively, according to manufacturers’ procedures (Invitrogen, Carlsbad, CA; 5 PRIME). AZI1 and EARLI1 expression in local, distal and untreated tissues was tested by 32-cycle PCR. Internal standard used for data normalization was EF1 α. Oligonucleotide sequences used as primers are presented in Supplementary Table 1 . Uncropped images from DNA gels are shown in Supplementary Fig. 9 . Subcellular localizations For localization studies in transgenic Arabidopsis carrying pBAV150:AZI1 construct, homozygous seedlings were sprayed with 30 μM Dex plus 0.1% Tween 20 solution and analysed by confocal microscopy 21 h later. For localization studies in N. benthamiana , A. tumefaciens C58C1 or LBA4404 strains harbouring the different constructs were infiltrated into leaves of 4-week-old plants. To express fusion proteins from pBAV150/154 vectors, 20 μM Dex solution was infiltrated onto leaves 1 day after agro-infiltration. Fractionation and confocal microscopy studies were done 21 h after Dex. For co-expression studies Agrobacterium harbouring different constructs were infiltrated together. Agrobacterium cultures were mixed immediately before infiltration. Arabidopsis cotyledons and N. benthamiana leaves were prepared as described [65] and a Zeiss LSM710 laser scanning confocal microscope (Zeiss, Germany) was used to visualize GFP fluorescence (excitation: 488 nm; emission: 505–530 nm), RFP fluorescence (excitation: 561 nm; emission: 570 to 620 nm) and chlorophyll autofluorescence (excitation: 633; emission: 650–750 nm). Images were taken using a LD C-Apochromat 40x/1.1 W Korr objective. Fluorescence in different channels was acquired for the same field using a sequential acquisition mode. For Z -series optical sections and time series video acquisition, images were taken at 512 × 512 pixels scanning resolution in maximum speed mode. Images, Z -series sections and time series videos were processed using ImageJ ( http://rsb.info.nih.gov/ij ), ZEN 2012 (Zeiss) and Adobe Photoshop software. ImageJ was also used for co-localization analysis and the generation of co-localizing pixels mask ( http://rsb.info.nih.gov/ij/plugins/colocalization.html ; thresholds=50% and ratio=75%). Fractionation To obtain microsomal fractions [66] , leaf tissue ( ∼ 1 g of N. benthamiana leaves) was frozen and ground in liquid nitrogen to a fine powder and then thawed in two volumes of ice-cold extraction buffer (50 mM Tris HCl, pH 7.5; 0.33 M sucrose; 5 mM EDTA; 150 mM NaCl and 1 × complete protease inhibitor cocktail from Roche). The crude extracts were filtered through two layers of Miracloth and centrifuged at 10,000 g for 10 min to get total protein extract (supernatant), which was further ultracentrifuged at 100,000 g for 60 min to get the microsomal membrane and soluble fractions, respectively. Membrane pellets were resuspended in extraction buffer or in buffers for membrane association strength analysis. Chloroplasts were isolated from 1 g of Arabidopsis or N. benthamiana leaves. Intact chloroplasts were purified using Percoll gradients [67] : homogenized leaves in Xpl buffer (0.33 M sorbitol, 50 mM HEPES pH 7.5, 2 mM EDTA, 1 mM MgCl 2 , 0.25% bovine serum albumin and 0.1% sodium ascorbate) were Miracloth-filtered, pelleted (2,000 g ) and resuspended to obtain a first total/impure chloroplast fraction. This fraction was layered on two Percoll gradients (40–80%) and centrifuged (9,000 g ) to purify the intact chloroplasts from the interphase boundary. Organelle purity was assessed by western blot using organelle-specific marker antibodies (see western blot analysis). To obtain apoplast extracts (intercellular washing fluid) [34] from N. benthamiana : fully expanded leaves of 4-week-old plants infiltrated with Agrobacterium harbouring the different constructs were vacuum infiltrated with sterile distilled water and leaf surfaces dried with absorbent paper before collection of the intercellular washing fluid. To collect the intercellular washing fluid, leaves were centrifuged in swinging buckets at 300 g for 15 min at 4 °C. Fluids were lyophilized before resuspension for use in western blots. Membrane association assay Membrane association assays [66] performed with microsomal protein extracts from N. benthamiana leaves infiltrated with Agrobacterium harbouring the different constructs. Extracts were treated with 1.5 M NaCl, 2 M urea, 1% Triton X-100, 1% NP-40+0.5% deoxycolate or 1% SDS, respectively, at 22 °C for 2 h with gentle shaking and fractionated into soluble supernatant or membrane pellet fractions by ultracentrifugation. Soluble fractions were precipitated by trichloroacetic acid before immunoblotting. Thermolysin protection assay Chloroplast fractions isolated from N. benthamiana leaves infiltrated with Agrobacterium harbouring the different constructs were treated with thermolysin [36] . Chloroplasts were resuspended in buffer (0.33 M sorbitol, 50 mM HEPES, pH 8) and thermolysin stock solution (1 mg ml − 1 thermolysin, 5 mM CaCl 2 , 0.33 M sorbitol, 50 mM HEPES, pH 8) added to give a final concentration of 0.1 mg ml − 1 thermolysin. Treated chloroplast were incubated for 30 min on ice, quenched by adding 10 mM EDTA and purified in a 40% Percoll cushion. Western blot analysis and immunoprecipitations Equal amounts of solubilized total (or different fractions) proteins were separated by SDS–polyacrylamide gel electrophoresis. Concentrations of protein extracts were measured by Bradford assay. Primary antibodies used for western blots were as follows: GFP antibody (Covance MMS-118P, 1:3,000; or Clontech cat. no. 632459, 1:3,000), HA antibody (Covance 16B12, 1:1,750), H + ATPase antibody (Agrisera AS07260, 1:7,500), cytosolic FBP antibody (Agrisera AS04 043, 1:3,000), BiP antibody (SPA-818, Stressgen, 1:3,000), ATPase β antibody [68] (1:3,000), DIR1 antibody [11] , [35] (1:20,000) and PR1 antibody [69] (1:3,000). For analysis of AZI1/EARLI1 native proteins from Arabidopsis an anti-EARLI1 polyclonal antibody [37] (that also recognizes AZI1) was used (1:750). The loading buffer for AZI1/EARLI1 western blot samples omitted reducing agents to allow detection of protein signals as described [37] . Secondary horseradish peroxidase-conjugated anti-rabbit or anti-mouse antibodies (Thermo Scientific) were used at 1:1,000. SuperSignal West Pico/Femto stable peroxidase (Thermo Scientific) was used to detect the signals. Gel-Pro analyzer software was used to quantify bands and Coomassie blue on western blots by densitometry. For immunoprecipitations, 1 g of N. benthamiana leaves were infiltrated with Agrobacterium harbouring the different constructs was used. Total extracts were isolated in two volumes of extraction buffer (50 mM Tris HCl pH 8.0, 10% glycerol, 0.5% sodium deoxycholate, 1% Igepal CA-630 from Sigma-Aldrich and complete protease inhibitor cocktail from Roche). Cellular debris was removed by Miracloth filtering, and 1 ml of supernatant was mixed with HA matrix (anti-HA affinity matrix, rat monoclonal 3F10, Roche) and incubated with gentle shaking at 4 °C ON. Matrix was then collected and washed 4–5 times with extraction buffer before resuspension in loading buffer for western blot analysis. Uncropped images from blot scans are shown in Supplementary Fig. 10 . Callose quantification Callose deposits were quantified according to Kim and Mackey [70] with some modifications. Leaves from six plants for each genotype/treatment were used for measurements. Water or 1 μM flg22 was infiltrated into Arabidopsis leaves 16–18 h before fixing in ethanol and staining with aniline blue (0.01% aniline blue in 150 mM K 2 HPO 4 , pH 9.5). Callose deposits were counted using ImageJ software from images taken with an epifluorescence microscope (Zeiss Axioskop, DAPI filter set). Data are shown as the number of deposits per 1.5 mm 2 . Protein alignment For AZI1 and DIR1 paralogs alignment ClustalW and BoxShade were used (EMBnet node Switzerland; http://www.ch.embnet.org/ ). Statistical analysis Analyses in this study were done with a statistical software package SigmaPlot v11.0 (Systat Software, Inc.). Analysis of variance (log-transformed data for bacterial growth curves) followed by the Newman–Keuls (SNK) post hoc test or one-tailed Student’s t -test were used as indicated in figure legends. How to cite this article: Cecchini, N. M. et al . Arabidopsis AZI1 family proteins mediate signal mobilization for systemic defence priming. Nat. Commun. 6:7658 doi: 10.1038/ncomms8658 (2015).